A network of molecular switches controls the activation of the two-component response regulator NtrC Recent successes in simulating protein structure and folding dynamics have demonstrated the power of molecular dynamics to predict the long timescale behaviour of proteins. Here, we extend and improve these methods to predict molecular switches that characterize conformational change pathways between the active and inactive state of nitrogen regulatory protein C (NtrC). By employing unbiased Markov state model-based molecular dynamics simulations, we construct a dynamic picture of the activation pathways of this key bacterial signalling protein that is consistent with experimental observations and predicts new mutants that could be used for validation of the mechanism. Moreover, these results suggest a novel mechanistic paradigm for conformational switching. Proteins involved in cellular signalling change their conformation in response to changes in environment (input signal), such as ligand binding or chemical modification, to control downstream cellular processes (output signal) [1] . The behaviour of these proteins is controlled by molecular level interactions between specific sets of residues that relay the signal. A detailed map of switches that facilitate conformational change has been obtained for only a few well-studied signalling proteins such as G-protein-coupled receptors and kinases [2] , [3] . We propose that atomistic simulations can help identify these key structural elements, and demonstrate this by examining the activation mechanism of nitrogen regulatory protein C (NtrC). This protein belongs to the family of two component regulatory systems ubiquitous in bacteria [4] , in which a phosphate is transferred from a sensor kinase (NtrB) to a response regulator (NtrC) [5] . This transfer activates the protein by triggering a structural rearrangement that exposes a hydrophobic surface and allows the protein to form oligomers essential for ATP hydrolysis [6] . Knowledge of the activation pathways and transition states of this rearrangement would be useful for elucidating new approaches for treating antibiotic-resistant infections. NtrC activation occurs when a phosphate is transferred from NtrB to D54 in NtrC. The active and inactive states are structurally very similar, with a root-mean-square deviation (RMSD) of only 2.9 Å (ref. 5 ). The inactive state is more flexible than the active state and could be described as a collection of states that rapidly interconvert [7] . The significant conformational change occurs in the region of residues 82–101, which is spatially removed from the phosphate-binding site at residue 54. The change involves a shift and slight uncoiling of helix 4 and minor rearrangement of the loop region between helix α 3 and beta-sheet β 3 (ref. 6 ). Recent nuclear magnetic resonance (NMR) studies have shown that both active and inactive states are populated in solution without phosphorylated D54, which demonstrates that phosphorylation is not required for the conformation change to occur [5] . Phosphorylation stabilizes the active state, which results in population inversion from a 2–10% active state population to 99% (ref. 8 ). Molecular simulations have been previously used to study conformational changes associated with NtrC. However, because of the large size of the protein and its long activation timescales, these studies have employed biased techniques such as targeted molecular dynamics [9] , separate simulations of the active and inactive states [7] , [10] , [11] , or simulations with coarse grained representations of the protein and solvent [12] , [13] , [14] , [15] . These studies have shed light on various aspects of NtrC activation but have failed to provide a comprehensive view of the conformational landscape of NtrC activation. In particular, kinetics of conformational transitions and detailed molecular description of NtrC activation pathways have not been reported. Understanding the activation mechanism of unphosphorylated NtrC is the focus of this study. We have employed enhanced sampling algorithms [16] coupled with the Folding@home [17] distributed computing platform to gather unprecedented statistics (1.6 ms) on NtrC dynamics for an atomistic description of the complex network of molecular-switches that drive activation of this key bacterial signalling protein. In this study, we use extensive MD simulations to build a Markov state model (MSM) for estimating the thermodynamics and kinetic properties of NtrC dynamics. MSMs reduce the complex conformational landscape of a protein to a set of metastable conformational states and the rates of transition between them [18] , [19] , [20] . The MSM of NtrC reveals a network of molecular switches that control NtrC activation and identifies metastable states on the NtrC conformational free energy landscape that could be targeted for inhibitor design. Simulations reveal molecular switches for NtrC activation MSMs for NtrC were built using snapshots along the simulated trajectories, and a 2,300 state MSM was chosen for analysis due to the convergence of its implied timescales, an indicator of Markovian behaviour (see Supplementary Fig. 1 and Methods). We started simulations from the inactive and active NMR structures of NtrC ( Fig. 1 ). A comparison of the MSM states reveals several residues that acquire distinct conformations and switch between different networks of interactions. In particular, we have identified four key ‘molecular switches’ that control NtrC activation as illustrated in Fig. 2a,b . The mechanism includes the F99 and Y94 switches, in which these residues rotate their side chains towards the protein core ( Fig. 3a,c ), the Y101–T82 switch that breaks its active state hydrogen bond ( Fig. 3b ) and the K67–Q96–Q95 (KQQ) switch ( Fig. 3d ), in which the K67–Q96 hydrogen bond breaks, destabilizing the C-terminal turn of helix α 4 , while a new hydrogen bond forms between K67 and Q95. Histograms of the residue pair distances that characterize the molecular switches were weighted by the MSM state equilibrium probability densities (see Methods) and are shown in Fig. 3a–d . The distributions reveal the bimodal nature of these switches and the overall activation process of NtrC. Although the solid line representing the sum of the state probabilities in Fig. 3a–d shows bimodal behaviour, the tail of the inactive state distribution extends into the active region due to greater conformational diversity in this state. This implies that the position of the switches alone is not sufficient to define the states and a kinetic definition of the active and inactive states (described below) must be used for understanding the activation mechanism. The probability density distributions also provide evidence against the commonly accepted theory related to the activation of response regulators such as NtrC and CheY [21] . In two-component systems like these, activation of the response regulator receiver domains has been proposed to rely on a ‘Y-T coupling’ mechanism [22] (Y101 and T82 in NtrC), where the interaction between this conserved pair of residues is correlated with the activation of the protein. Figure 3b shows the probability distributions of Y101–T82 distance in the active, inactive and entire conformational ensemble of NtrC. The active ensemble shows two peaks corresponding to conformations with Y-T coupling formed and broken. 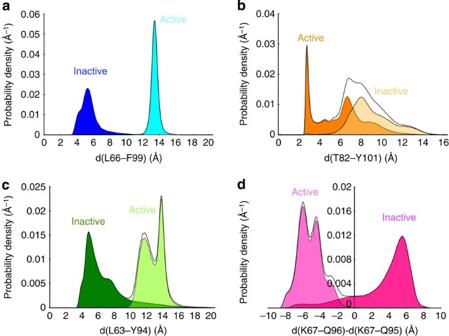Figure 3: Thermodynamics of molecular switches. MSM state population weighted probability densities of (a) L66–F99 distance, (b) T82–Y101 distance, (c) L63–Y94 distance and (d) difference between K67–Q96 and K67–Q95 distances (shown separately inSupplementary Fig. 2). The different colour shades correspond to the different kinetically defined states, whereas the solid line represents the entire data set. This figure provides the evidence that the Y101–T82 coupling can be either formed or broken within the active state, but is predominately broken in the inactive state. This result implies that Y-T coupling is not strictly correlated with the activation of NtrC and is in agreement with recent NMR relaxation dispersion experiments [10] , which found the interconversion of the Y101 rotameric state to be faster than the inactive/active conformational transition. Furthermore, our results in Fig. 3a,c,d indicate that the conformational preferences of the three switches identified in this study involving F99, Y94 and the KQQ residues are more strongly correlated with activation than Y-T coupling. In particular, the slowest dynamical process of the MSM (see Methods and Supplementary Figs 2–4 ) involves the flipping of the KQQ switch identified in this study, which underscores its importance in NtrC activation. These results also show that these couplings or switches could be either formed or broken within active or inactive ensemble. 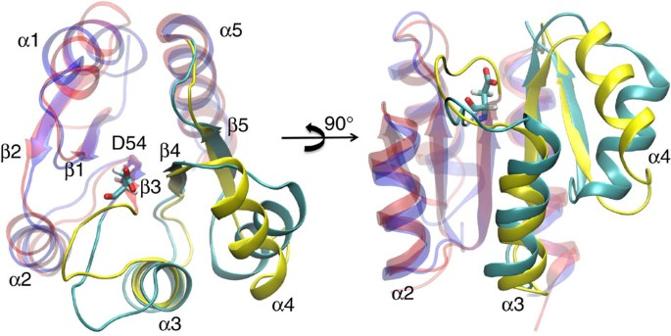However, the probability of toggling of individual switches is dependent on the overall state of the protein. Figure 1: Conformational changes associated with NtrC activation. The active (blue; cyan) and inactive (red; yellow) crystal structures of NtrCr with the regions involved in conformational switching highlighted in cyan (active) and yellow (inactive). The phosphorylation of residue D54 shown above involves large structural changes in and around helixes 3 and 4. Figure 1: Conformational changes associated with NtrC activation. The active (blue; cyan) and inactive (red; yellow) crystal structures of NtrCr with the regions involved in conformational switching highlighted in cyan (active) and yellow (inactive). 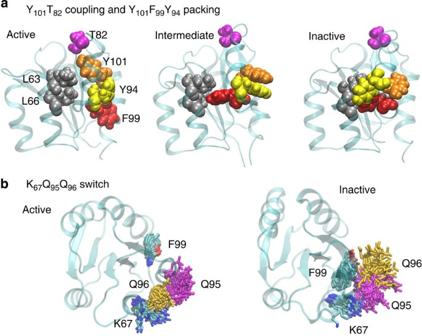The phosphorylation of residue D54 shown above involves large structural changes in and around helixes 3 and 4. Figure 2: Molecular switches involved in NtrC activation. (a) Changes in T82–Y101 coupling and changes in hydrophobic packing between residues L63, L66, Y94, F99 and Y101 during activation. (b) Switching of interaction partner of K67 from Q96 in active state to Q95 in inactive state. Full size image Figure 2: Molecular switches involved in NtrC activation. ( a ) Changes in T82–Y101 coupling and changes in hydrophobic packing between residues L63, L66, Y94, F99 and Y101 during activation. ( b ) Switching of interaction partner of K67 from Q96 in active state to Q95 in inactive state. Full size image Figure 3: Thermodynamics of molecular switches. MSM state population weighted probability densities of ( a ) L66–F99 distance, ( b ) T82–Y101 distance, ( c ) L63–Y94 distance and ( d ) difference between K67–Q96 and K67–Q95 distances (shown separately in Supplementary Fig. 2 ). The different colour shades correspond to the different kinetically defined states, whereas the solid line represents the entire data set. Full size image Identifying intermediate states of NtrC We identify several metastable intermediate states along the activation process that are characterized by the toggling of individual switches between their active and inactive conformations. In the active state of NtrC, hydrophobic residues Y94, F99 and Y101 form a solvent-exposed hydrophobic surface ( Fig. 2a ). Breakage of the Y101–T82 hydrogen bond and rotation of the F99 side chain triggers collapse of this exposed hydrophobic surface, and these residues switch to their inactive conformations, directed towards the protein core. These conformational changes are coupled to the exchange of K67 interaction partners, from Q96 to Q95 ( Fig. 2b ) via switching of the Y94 side chain. The K67–Q96 interaction is disrupted, followed by formation of the K67–Q95 contact and flipping of Y94 towards the protein core. This KQQ conformational switch motif defines several key intermediate states, mapped onto the activation landscape in Fig. 4b , and is enabled by changes in the fold of helix during activation. 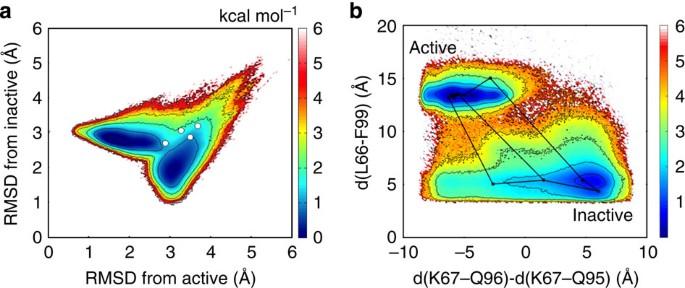Figure 4: NtrC activation pathways. Contour plots of (a) RMSD of NtrC from active and inactive states, (b) distance between Cαatoms of the L66–F99 residues versus the difference in distance between K67–Q96 and K66–Q95. MSM states with committor values between 0.2 and 0.8 are shown as white circles. The black lines show the three top pathways calculated from transition path theory. Figure 4: NtrC activation pathways. Contour plots of ( a ) RMSD of NtrC from active and inactive states, ( b ) distance between C α atoms of the L66–F99 residues versus the difference in distance between K67–Q96 and K66–Q95. MSM states with committor values between 0.2 and 0.8 are shown as white circles. The black lines show the three top pathways calculated from transition path theory. Full size image Role of transient hydrogen bonds in activation Our results reveal a hydrogen bond network exchange that allows partial unfolding and refolding of helix α 4 to accommodate the conformational rearrangement of the hydrophobic surface residues. During activation, the helix α 4 C-terminal end gains two backbone hydrogen bonds (between V91–Q95 and S92–Q96 ( Supplementary Fig. 5 )) and loses two backbone hydrogen bonds (between H84–D88 and S85–A89 ( Supplementary Fig. 6 )) because of the formation of a helix turn at its N-terminal end. Gardino et al. [23] have shown that residues S85 and D86 ( Supplementary Fig. 7 ) at the N-terminal side of helix 4 and residues Q96 and Y101 at the C-terminal side of helix α 4 and beta-sheet β 5 , respectively, form transient hydrogen bonds that compensate for the loss of backbone hydrogen bonds and lower the energy barrier for activation. The MSM-derived thermodynamic populations and exchange kinetics between states with these transient hydrogen bonds reveal that the S85–D86 hydrogen bonds ( Supplementary Figs 8 and 9 ) are formed both in the inactive and active state ensemble in our simulations, not just in the transition state. This indicates that a more complex mechanism is responsible for slow inter-conversion rate of S85D and S85G mutants reported by Gardino et al. [24] , and fast inter-conversion rate of S85N mutant. Similarly, the transient Y101–Q96 hydrogen bond is also found to be well-formed in the inactive state ( Supplementary Figs 8 and 9 ) becaue of fluctuations of the unfolded, C-terminal half turn of helix α 4 . Gardino et al. [23] have shown that both the Q96N and the Y101F mutants of NtrC have a slower inter-conversion rate between active and inactive states (≈3,500 versus 13,300 s −1 for wild type). The residues Q96 and Y101 interact with different hydrogen bond partners forming T82–Y101, K67–Q96 and Y101–Q96 hydrogen bonds in different conformations ( Fig. 2a,b ). The substitutions Y101F and Q96N not only affect the transition state stability but also the active/inactive states. Therefore, it is difficult to provide a rational mechanistic explanation of the slow interconversion rate observed in experiments and further computational investigations are needed to obtain an atomistic perspective of the effect of these substitutions. Diverse activation pathways due to heterogeneity in basins The MSM-weighted two-dimensional contour plots of the simulation data are plotted in Fig. 4a as the backbone atom RMSD from both active and inactive states and Fig. 4b as the K67–Q95–Q96 and L66–F99 switch distances. Both plots clearly show two dominant basins, reinforcing our view that both states are populated even without the presence of the activating phosphate group. The plots show that these limited structural features alone are insufficient to characterize the inactive and active states. MSM-derived ‘committor’ values and high-flux pathways between the active and inactive states were computed (see Methods and Supplementary Fig. 3 ), and states with intermediate committor values are shown as white circles in Fig. 4 to represent transition states with similar probability of transitioning forward to the active state or backward to the inactive state. These states lie around the edges of the inactive basins in both plots, yet they have a 20–80% probability of transitioning into the active basin instead of returning to the inactive basin. Our MSM approach allows us to define states by their kinetic connections and reveal their role in the activation mechanism, instead of relying on structural differences that can be difficult to elucidate. We can, however, structurally characterize these kinetic intermediate states in terms of the previously described molecular switches and we find that several kinetic intermediate states are present along the activation pathways. For example, the basins in the contour plot for the K67–Q95–Q96 and L66–F99 switch distances ( Fig. 4b ) are connected by multiple pathways with different kinetic intermediates depending on which switch is toggled first [12] . The highest flux pathway involves the kinetic intermediate state, where KQQ switch is toggled before the F99 flip ( Supplementary Fig. 10 ). Similarly, kinetic intermediates along the activation pathways could be identified with differences in the state of molecular switches. The top three activation pathways reveal kinetic intermediates with L63-Y94 switch toggled before KQQ flip ( Supplementary Fig. 11 ) and L63–Y94 switch toggled before the F99 flip. One of the key debates about the NtrC activation mechanism centres on the requirement for cracking, which is defined as a complete unfolding of helix α 4 for the activation conformational transition [9] , [12] . Although we have seen an exchange of hydrogen bond networks involving this helix, as described above, our activation pathway results do not show a cracked helix α 4 . Similarly, ultra-long trajectories generated from a kinetic Monte Carlo simulation using the MSM state transition probabilities ( Fig. 5a ) show that the Solvent Accessible Surface Area of helix α 4 increases slightly in the inactive state because of the rotation of the helix, which is also in agreement with previous NMR results [23] , [24] . The increase in the Solvent Accessible Surface Area would be much higher ( ∼ 2,600 Å 2 ) for the fully unfolded helix α 4 . 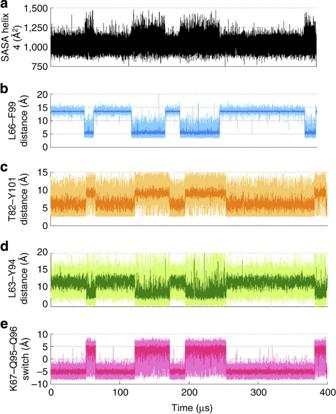Figure 5: Kinetics of molecular switches. Variation of the order parameters (a)α-helicity of helixα4and distance between (b) L66–F99, (c) T82–Y101, (d) L63–Y94 and (e) the difference of (K67–Q96) and (K67–Q95) residues along a MSM trajectory generated using a kinetic Monte Carlo algorithm and MSM state transition probabilities. The light colour represents the instantaneous value along the trajectory, whereas the dark shade is a moving average over ten frames. Figure 5: Kinetics of molecular switches. Variation of the order parameters ( a ) α -helicity of helix α 4 and distance between ( b ) L66–F99, ( c ) T82–Y101, ( d ) L63–Y94 and ( e ) the difference of (K67–Q96) and (K67–Q95) residues along a MSM trajectory generated using a kinetic Monte Carlo algorithm and MSM state transition probabilities. The light colour represents the instantaneous value along the trajectory, whereas the dark shade is a moving average over ten frames. Full size image Kinetics of NtrC activation The activation and deactivation timescales (mean first passage time between inactive and active micro states) are found to be 90 and 110 μs, respectively, which are in agreement with the experimental interconversion rate of 77 μs (ref. 24 ). A visual inspection of the kinetic plots ( Fig. 5b–e ) suggests that a single thermal fluctuation toggles all the molecular switches via a concerted mechanism, where molecular switches are triggered cooperatively. However, the conformational landscape of molecular switches in Fig. 3 and Supplementary Figs 10–12 indicate a different, more sequential view of NtrC activation, where a particular molecular switch is turned on or off before other switches change their conformation (as described above). Altogether, these results indicate that several switches are required to toggle their states before crossing the final barrier to activation/deactivation and they become locked in that state after the barrier is crossed. For example, the Y101–T82 switch toggles between the on and off state in active basin but it is always broken after crossing the deactivation barrier ( Fig. 3b ). Similar observations can be made for the L63–Y94 and KQQ switches ( Supplementary Figs 10–12 ). Figure 5c,d shows that the Y101–T82 and L63–Y94 distances fluctuate between two distinct states but the instantaneous value of these fluctuations (light colour) overlap with the average values (dark colour). This means that these switches are not a strong indicator of state because the instantaneous value of the order parameter does not give any state information. This gives further evidence for our hypothesis that ‘Y-T coupling’ is not strictly correlated with the activation of NtrC. Figure 5b,e shows agreement between the instantaneous value and the average value indicating that the KQQ switch distinguishes the active and inactive states and further implicates this switch as the rate-limiting step. Finally, the equilibrium population of the active ( ρ active ∼ 0.16) and inactive state ( ρ inactive ∼ 0.09) indicate that both states are populated in solution and interconvert rapidly at the simulation temperature (340 K), with a barrier between intermediate and inactive states ∼ 4 kcal mol −1 as estimated from the free energy contour plots ( Fig. 4 ). The predicted barrier height between the intermediates and inactive state is 4–5 kcal mol −1 , which, when allowing for temperature change, is close to the reported 6 kcal mol −1 activation barrier measured experimentally using NMR at 300 K (ref. 23 ). Our results contribute to the prominent debate about conformational change mechanisms in general, comparing a sequential domino brick effect [25] or Monod-Wyman-Changeux [25] , [26] , [27] type of concerted action allostery. For NtrC activation, we find that the molecular switches are all connected (a requirement for the domino effect) and can induce a sequential triggering of switches, such as T82-Y101 hydrogen bond breakage preceding rearrangement of the hydrophobic surface. However, we also observe that the KQQ motif and Y94 switch their conformations cooperatively. The sequential flipping of these residues occurs within the lag time of the model so it appears concerted in the kinetic plots in Fig. 5 . Therefore, the mechanism of global conformational change associated with NtrC activation lies between a sequential and cooperative mode of molecular switching so that the system is ‘functionally concerted’. MSMs provide a third and more natural framework for understanding complex conformational changes in proteins. MSMs provide a probabilistic network-switching model where different molecular switch conformations are represented by discrete MSM states and the rate of transition between these states accounts for both the independent switch probability and the conditional probability of a switch toggle given the states of other switches. An important advantage of this discrete probabilistic picture of global conformational change is that it allows characterization of both sequential switching and concerted conformational change, depending on the time resolution needed to understand a particular mechanism. Comparing this study to recent work in the Kern group [28] illustrates the robustness of MSMs for interpreting conformational change. Kern’s work used CHARMM force field instead of amber99sb, which caused an increase in conformational heterogeneity, especially in the inactive state. Also, the Kern study started from several structures along the activation pathway based on a targeted molecular dynamics (TMD) trajectory [9] , whereas the present study used unbiased molecular dynamics (MD) and adaptive sampling. In general, string methods allow sampling of long processes with less computation time than corresponding unbiased methods but increases the risk of discovering unphysical results. In this case, the string method of seeding states along the activation pathway allowed the Kern group to identify an inactive state in better agreement with recent NMR, where F99 is correctly facing helix 3. Despite these notable differences in methodology, the major conclusions were in agreement with: the inactive is a collection of states interconverting rapidly, there are multiple activation pathways connecting the basins, and a kinetic, rather than structural, state definition is required to differentiate states. A more complete discussion including comparison figures can be found in the Kern study [28] . In summary, we have obtained a detailed atomistic view of the conformational transition of the key bacterial signalling protein, NtrC. The mechanistic insights obtained from this study suggest newly recognized molecular switches that play a central role in NtrC activation, such as the KQQ and Y94 switches. These results also suggest that residues far from the activating phosphorylation site and output domain play an important role in activation. The influence of such residues, such as K67, L66 and L63, could be validated using NMR and other spectroscopic methods. The results presented here also support a mechanism in which phosphorylation of D54 would lock the protein in active state, consistent with other work on this system [6] . Hydrogen bonding between phosphate group at D54, which is in proximity to the hydroxyl group of T82, would stabilize the Y101–T82 switch, which we observe to fluctuate without the presence of phosphate, and lock the entire protein in active state. MSMs have been used extensively to study large-scale conformational changes involved in protein folding as well as more subtle changes involved in receptor activation and ligand binding [29] , [30] , [31] , [32] , [33] , [34] , [35] , [36] . This study further supports the utility of MSMs as a natural framework for understanding and quantifying changes in hydrogen bond networks or residue side chain rotations associated with many protein conformational changes in signalling networks. Furthermore, these results indicate that in silico approaches [20] combined with advances in computer hardwares [37] can be used successfully and routinely for obtaining mechanistic understanding of cellular signalling phenomena. Simulation details The starting structures for these simulations are the end result of a series of modelling procedures applied to the NMR structures 1DC7 and 1DC8 (ref. 5 ). In addition to the refinement described by Lei et al. [9] , helix 3 was completed and helix 4 was extended by two residues in order to match dihedral and distance constraints. The isomeric state of P104 has also been corrected. The structures were then parameterized using CHARM27 (ref. 38 ) with cross-term energy correction map (CMAP) correction [39] , solvated in TIP3P water [40] , and neutralized with sodium ions. Nanoscale molecular dynamics (NAMD) [41] was used to minimize the structure with a series of conjugate gradients, gradually releasing constraints from the protein. Heating was performed in the NVT (canonical) ensemble, gradually increasing the temperature from 50 to 300 K in increments of 25 K and simulating each step for 50 ps with a time step of 1 fs. Hydrogen atoms were constrained using SHAKE (Gauss-Seidel method which approximates the solution of the linear system of equations) [42] , and a non-bonded cutoff of 14 Å was used. The simulation was continued at 300 K in the NPT ensemble using Langevin dynamics with a time step of 2 fs, a damping coefficient of 5 per ps and a non-bonded cutoff of 12 Å. Pressure was controlled with a Nose-Hoover [43] piston with a 200-fs period of oscillation and a damping time of 100 fs. Electrostatics were computed using PME10 with a grid size of 72 × 72 × 72 Å 3 , a direct space tolerance of 10 −6 and an interpolation order of 6. The two initial structures were placed in a dodecahedron box with radius 10 Å from the proteins (edge length 75 Å) and solvated in 8,000 TIP3P water molecules. The system was then relaxed using a steepest decent algorithm using the Amber99SB [44] forcefield in the simulation package GROMACS 4.5 (ref. 45 ) for 500 steps with step size 1 fs. Next, the structures were equilibrated with restrained all protein atom positions for 100 ns with all bonds constrained using linear constraint solver (LINCs) [46] . The equilibration used Berendsen pressure coupling with time constant of 1 ps, compressibility 4.5 × 10 −5 and reference pressure 1 bar and the v-rescale temperature coupling to 300 K. Note that in GROMACS, the v-rescale option is velocity rescaling with a stochastic term, which ensures a canonical ensemble [47] . The two equilibrated structures were used to start 30,000 parallel simulations on the distributed computing network Folding@home. These simulations used a 2-fs time step and a grid-based neighbour list was updated every 10 steps with a 10-Å cutoff. All bonds were again constrained using LINCS [46] with two iterations to fourth order. Production runs were done in the NVT ensemble using v-rescale [47] to maintain system temperature of 300 K. Coulombic and van der Waals interactions were switched off between 8 and 8.4 Å. Linear centre of mass motion was removed every step. Random initial velocities were drawn from a Maxwell-Boltzmann distribution at 300 K. After collecting 250 μs of aggregate data, the data from each conformation were clustered at an RMSD cutoff of 1.25 Å to generate a 6,838 state model for the active state and a 14,232 state model for the inactive state for a round of adaptive sampling [16] . Conformations representing the state centres were used to start additional simulations. In addition to the adaptive sampling, 15,000 new simulations were started from the active and the inactive conformations at a slightly increased temperature of 340 K in order to more quickly sample conformational space. In total, 7,917,355 snapshots were stored in increments of 0.2 ns totaling 1,582 μs of data. All protein structures were rendered in visual molecular dynamics (VMD) [48] and figures created using Matplotlib [49] with the Numpy [50] scientific computing package. Markov state models MSMs use discrete time master equations models to map out molecular conformational space [33] , [51] . Atomistic molecular dynamics simulations are first clustered based on geometric similarity, then kinetic information is used to group conformations that interconvert rapidly into metastable states. MSMs allow more automated simulation analysis that relies less on human intuition, an advancement over previous techniques. MSMs have been used to make direct connections from simulations to experiments, such as ab initio structure prediction for the villin headpiece and characterization of its conformational dynamics [52] , [53] , [54] . The MSMbuilder 2.5 package [55] was used to construct a microstate model with 2,314 states. The microstate model was generated by clustering conformations at 2 ns intervals using the RMSD of all backbone heavy atoms as a metric and the k-centres clustering algorithm, followed by ten iterations of the local k-medoids algorithm, with a 2.25-Å RMSD cutoff. The remaining 90% of the data were then assigned to these clusters and used to construct a transition probability matrix. A second clustering based on 25% of the data gave a very similar state decomposition, which suggests the system is well sampled. Maximum Likelihood Estimator [18] was used to generate a transition probability matrix T ij , which maps out the probability of transitioning from state i at time t to state j at time t + τ , where τ is the lag time of the model. The Markov lag time is the time interval with demonstrated Markovian behaviour and can be determined by plotting the implied time scales ( k ) from eigenvalues μ of the transition probability matrix at varied lag times τ as k =− τ / ln ( μ ). The implied timescales should converge to an unchanged rate when Markovian behaviour is achieved, which corresponds to 4 ns for NtrC ( Supplementary Fig. 1 ) [56] . The first and second eigenvectors of the transition probability matrix T ij provide, respectively, the equilibrium conformational state populations and the slowest dynamical process on the conformational landscape. MSM-weighted probability distributions, both one- and two-dimensional, are obtained by binning the raw data within each MSM state and weighting it by the MSM equilibrium state population. High-flux pathways between active and inactive states and MSM state committor values are also calculated from T ij using the transition matrix definition of transition path theory [57] , [58] . Committor values measure the probability of reaching the active state (at values near one) before returning to the inactive state (at values near zero). Intermediate committor values near 0.5 represent transition states capable of transitioning either back to inactive state or forward to the active state. How to cite this article: Vanatta, D. K. et al. A network of molecular switches controls the activation of the two-component response regulator NtrC. Nat. Commun. 6:7283 doi: 10.1038/ncomms8283 (2015).